Cleavage and nuclear localization of the rice XA21 immune receptor Plants and animals carry specific receptors that recognize invading pathogens and respond by activating an immune response. The rice XA21 receptor confers broad-spectrum immunity to the Gram-negative bacterial pathogen, Xanthomonas oryzae pv. oryzae upon recognition of a small protein, Ax21, that is conserved in all Xanthomonas species and related genera. Here we demonstrate that XA21 is cleaved to release the intracellular kinase domain and that this intracellular domain carries a functional nuclear localization sequence. Bimolecular fluorescence complementation assays indicate that the XA21 intracellular domain interacts with the OsWRKY62 transcriptional regulator exclusively in the nucleus of rice protoplasts. In vivo cleavage of XA21 and translocalization of the intracellular kinase domain to the nucleus is required for the XA21-mediated immune response. These results suggest a new model for immune receptor function: on receptor recognition of conserved microbial signatures, the associated kinase translocates to the nucleus where it directly interacts with transcriptional regulators. Plants and animals perceive conserved microbial signatures via plasma membrane and cytoplasmically localized receptors [1] . Such immune receptors, also called pattern recognition receptors, include animal TLRs (Toll-like receptors) and plant receptor kinases (RKs). These receptors often carry serine-threonine kinases of the non-arginine aspartate (non-RD) class that are either integral to the receptor (plants) or associated with it (animals) [2] , [3] . Whereas RD kinases are regulated by autophosphorylation of the activation segment, a centrally located loop that sits close to the catalytic centre, very little is known about non-RD kinase activation. In plants, well-studied immune receptors that carry the non-RD kinase motif include rice XA21 ( Xanthomonas resistance 21), Arabidopsis FLS2 (flagellin sensitive 2) and the Arabidopsis elongation factor Tu receptor (EFR). All plant RKs characterized to date that carry the non-RD kinase motif are involved in recognition of conserved microbial signatures [2] . Animal immune receptors include TLR1, 3, 5, 6, 7, 8 and 9, which signal via non-RD interleukin-1 receptor-associated kinases 1 (IRAK1), and TLR3 and TLR4, which signal through non-RD receptor interacting protein 1 kinases [1] , [3] , [4] . A general theme that has emerged from these studies is that non-RD kinase activity is at least partially dispensable for the innate immune response in both plants and animals [1] and that the kinases function partly as phosphorylation-mediated scaffold proteins that recruit different signaling components [4] . In rice, the XB24 ATPase physically associates with the XA21 juxtamembrane domain and uses ATP to promote phosphorylation of certain Ser/Thr sites on XA21, keeping the XA21 protein in an inactive state [5] . Together these results suggest that non-RD kinases are activated in a manner distinctly different from the well-characterized RD kinases. Similar to the plant immune receptors, all members of the epidermal growth factor receptor (EGFR) family have an extracellular ligand-binding domain, a transmembrane domain, and a cytoplasmic kinase domain. Many of these receptors require a nuclear translocation step for their signal transductions. For example, in response to binding their corresponding ligands, the intact protein or the intracellular domain of the EGFR family members, ErbB-1 (v-erb-a erythroblastic leukemia viral oncogene homologue 1), ErbB-2, ErbB-3 and ErbB-4 are translocated to the nucleus [6] , [7] . ErbB-2 and ErbB-4 carry proline-rich carboxyl termini that contain intrinsic transcription activity and function as transcriptional regulators in the nucleus [8] , [9] , [10] . ErbB-1 interacts with the transcription factors STAT3 (signal transducer and activator of transcription 3), STAT5 and E2F transcription factor-1. Each of these transcription factors then regulates expression of target genes [11] , [12] , [13] . Such nuclear translocation events have not been reported for receptor kinases governing the innate immune response. Here we show that XA21 is cleaved to release the intracellular kinase domain and that this intracellular domain carries a functional nuclear localization sequence. Bimolecular fluorescence complementation (BiFC) assays indicate that the XA21 intracellular domain interacts with the OsWRKY62 transcriptional regulator exclusively in the nucleus of rice protoplasts. In vivo cleavage of XA21 and translocalization of the intracellular kinase domain to the nucleus is required for the XA21-mediated immune response. These results suggest a new model for immune receptor function where, upon receptor recognition of conserved microbial signatures, the associated kinase translocates to the nucleus and directly interacts with transcriptional regulators. XA21 is cleaved to release the intracellular kinase domain Rice XA21 confers immunity to the Gram-negative bacterium Xanthomonas oryzae pv. oryzae ( Xoo ) [14] , XA21 binds a conserved sulphated peptide, called AxY S 22 derived from the Xoo Ax21 (activator of XA21-mediated immunity) protein [15] . We previously reported that on binding to AxY S 22, XA21 accumulates, releasing a 110-kDa amino-terminal cleavage product in transgenic rice plants expressing a N-terminal Myc-tagged XA21 (Myc-XA21) [15] , [16] , [17] . Here we show that a 70-kDa carboxy-terminal cleavage product, corresponding to the kinase domain fused to cyan fluorescent protein (CFP), is also detected after infection of transgenic rice plants carrying a C-terminal CFP-tagged XA21 (XA21-CFP) [18] ( Supplementary Fig. S1 and Fig. 1 ). To further characterize the XA21 cleavage product, we used rice lines expressing Myc-XA21 [18] and XA21-CFP [18] . A 110-kDa N-terminal cleavage product was immunoprecipitated using an agarose-conjugated anti-Myc antibody. This 110 kDa product did not cross-react with the anti-XA21 kinase antibody ( Fig. 1a ). The 70-kDa C-terminal cleavage product immunoprecipitated using the anti-green fluorescent protein (GFP) antibody did not react with the anti-XA21 LRR antibody ( Fig. 1b ). These results indicate that 110 kDa C-terminal cleavage product consists of the XA21 intracellular domain. 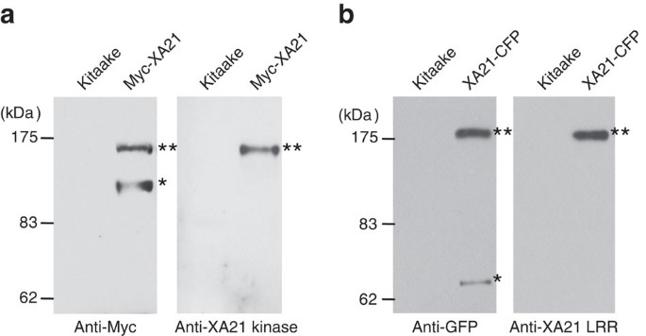Figure 1: XA21 cleavage releases the intracellular kinase domain. (a) Protein extracts from Kitaake and Myc-XA21 (T4, 20-4-2) plants were immunoprecipitated with agarose-conjugated anti-Myc antibody. The immunoprecipitates were separated on duplicate gels and transferred to membranes for western blot analysis. Two bands were detected using anti-Myc antibody (left) and a single band was detected using anti-XA21 kinase antibody (right). The upper 140 kDa band (marked with '**') corresponds to the full-length Myc-XA21 fusion protein and the lower 110 kDa band (marked with '*') corresponds to the N-terminal cleavage product15,16,17,42. (b) Protein extracts from Kitaake and XA21-CFP (T3, 15A-1-1-4) plants were immunoprecipitated with agarose-conjugated anti-GFP antibody. The immunoprecipitates were separated on duplicate gels and transferred to membranes for western blot analysis. Two bands were detected using anti-GFP antibody, (left) and one band was detected using anti-XA21 LRR antibody (right). The upper 180 kDa band (marked with '**') corresponds to the full-length XA21-CFP fusion protein. The lower 70 kDa band (marked with '*') corresponds to the C-terminal cleavage product. Figure 1: XA21 cleavage releases the intracellular kinase domain. ( a ) Protein extracts from Kitaake and Myc-XA21 (T 4 , 20-4-2) plants were immunoprecipitated with agarose-conjugated anti-Myc antibody. The immunoprecipitates were separated on duplicate gels and transferred to membranes for western blot analysis. Two bands were detected using anti-Myc antibody (left) and a single band was detected using anti-XA21 kinase antibody (right). The upper 140 kDa band (marked with '**') corresponds to the full-length Myc-XA21 fusion protein and the lower 110 kDa band (marked with '*') corresponds to the N-terminal cleavage product [15] , [16] , [17] , [42] . ( b ) Protein extracts from Kitaake and XA21-CFP (T 3 , 15A-1-1-4) plants were immunoprecipitated with agarose-conjugated anti-GFP antibody. The immunoprecipitates were separated on duplicate gels and transferred to membranes for western blot analysis. Two bands were detected using anti-GFP antibody, (left) and one band was detected using anti-XA21 LRR antibody (right). The upper 180 kDa band (marked with '**') corresponds to the full-length XA21-CFP fusion protein. The lower 70 kDa band (marked with '*') corresponds to the C-terminal cleavage product. Full size image The XA21 intracellular kinase translocates to the nucleus To localize the XA21 intracellular domain in vivo , we investigated the cellular distribution of C-terminal GFP-tagged XA21 (XA21-GFP) in rice protoplasts. Consistent with our previous results [16] , XA21-GFP is localized both to the plasma membrane and the cortical and perinuclear endoplasmic reticulum in the absence of AxY S 22 ( Fig. 2a and Supplementary Fig. S2 ). GFP alone localizes to both the nucleus and cytoplasm ( Supplementary Fig. S3a ). In contrast, treatment with AxY S 22 ( Fig. 2a ) or with supernatants prepared from Xoo [15] ( Supplementary Figs S2 and S4 ) triggers significant accumulation of the XA21-GFP inside the nucleus (24.1±3.8% of the protoplasts accumulated XA21-GFP protein in the nucleus, Supplementary Table S1 ). Nuclear localization was not observed in protoplasts treated with water or the biologically inactive peptide, AxY22 [15] . (1.2±0.1% and 1.8±0.7%, respectively; Fig. 2a and Supplementary Table S1 ). These results indicate that the XA21 intracellular domain translocates to the nucleus in protoplasts after treatment with biologically active AxY S 22. 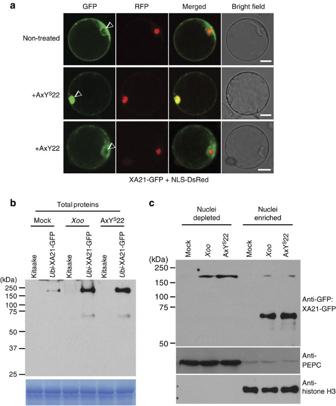Figure 2: Nuclear translocation of XA21-GFP after treatment with AxYS22 peptide orXoo. (a) XA21-GFP was expressed in rice protoplast cells using polyethylene glycol-mediated transformation. AxYS22 or AxY22 peptides were applied 16 h after transformation. Expression of the introduced genes was observed 1 h after peptide treatment. NLS-DsRed (nuclear localization signal-Discosomasp. red fluorescent protein) was co-transformed as a nucleus marker. Images were collected using a Leica True Confocal Scanner SPE confocal microscope and coded in green and red for GFP and DsRed, respectively. Two confocal z-section images were merged to have a 2D image. Arrowheads mark the nuclei. Scale bar, 10 μm. (b) Western blot analysis of XA21-GFP proteins extracted from transgenic rice plants expressingXA21-GFPunder the control of theUbipromoter (Ubi-XA21-GFP, homozygous 5-5-4). Equal amount of total proteins (75 μg) were extracted from leaf discs of Kitaake andUbi-XA21-GFP plants 3 h after Mock,Xooor AxYS22 treatment. XA21-GFP and C-terminal cleavage product, detected with an anti-GFP antibody, displayed bands of approximately 170 and 70 kDa, respectively. Equal loading of total proteins was confirmed by Coomassie blue staining of proteins (lower panel). (c) Western blot analysis of XA21-GFP extracted from nuclei-depleted and nuclei-enriched fractions fromUbi-XA21-GFP line (homozygous 5-5-4) detected by the anti-GFP antibody. Nuclei-enriched (100 μg) and nuclei-depleted (100 μg) fractions were prepared from total proteins inb. XA21-GFP and C-terminal cleavage product-GFP displayed bands at approximately 170 and 70 kDa, respectively. Cytolsolic phosphoenolpyruvate carboxylase (PEPC) and nuclear histone H3 protein were used as cytosolic and nuclear markers, respectively. Figure 2: Nuclear translocation of XA21-GFP after treatment with AxY S 22 peptide or Xoo . ( a ) XA21-GFP was expressed in rice protoplast cells using polyethylene glycol-mediated transformation. AxY S 22 or AxY22 peptides were applied 16 h after transformation. Expression of the introduced genes was observed 1 h after peptide treatment. NLS-DsRed (nuclear localization signal- Discosoma sp. red fluorescent protein) was co-transformed as a nucleus marker. Images were collected using a Leica True Confocal Scanner SPE confocal microscope and coded in green and red for GFP and DsRed, respectively. Two confocal z-section images were merged to have a 2D image. Arrowheads mark the nuclei. Scale bar, 10 μm. ( b ) Western blot analysis of XA21-GFP proteins extracted from transgenic rice plants expressing XA21-GFP under the control of the Ubi promoter ( Ubi -XA21-GFP, homozygous 5-5-4). Equal amount of total proteins (75 μg) were extracted from leaf discs of Kitaake and Ubi -XA21-GFP plants 3 h after Mock, Xoo or AxY S 22 treatment. XA21-GFP and C-terminal cleavage product, detected with an anti-GFP antibody, displayed bands of approximately 170 and 70 kDa, respectively. Equal loading of total proteins was confirmed by Coomassie blue staining of proteins (lower panel). ( c ) Western blot analysis of XA21-GFP extracted from nuclei-depleted and nuclei-enriched fractions from Ubi -XA21-GFP line (homozygous 5-5-4) detected by the anti-GFP antibody. Nuclei-enriched (100 μg) and nuclei-depleted (100 μg) fractions were prepared from total proteins in b . XA21-GFP and C-terminal cleavage product-GFP displayed bands at approximately 170 and 70 kDa, respectively. Cytolsolic phosphoenolpyruvate carboxylase (PEPC) and nuclear histone H3 protein were used as cytosolic and nuclear markers, respectively. Full size image To investigate whether the XA21 intracellular domain translocates to the nucleus in mature plants, we generated stable transgenic rice plants expressing biologically active XA21-GFP ( Ubi -XA21-GFP, Supplementary Fig. S5 ; Native -XA21-GFP, Supplementary Fig. S6 ). After Xoo infection or AxY S 22 treatment of Ubi -XA21-GFP plants, the XA21-GFP protein accumulates ( Fig. 2b ). This result is consistent with our published studies showing that Xoo treatment triggers enhanced XA21 protein accumulation without a corresponding increase in transcription [16] . We also observed a significant increase of the XA21 intracellular domain in the nuclei-enriched fraction ( Fig. 2b,c , and Supplementary Fig. S7 ). In contrast, the intracellular domain was not detected in nuclei-enriched fractions after mock infection. These results indicate that AxY S 22 recognition triggers accumulation of XA21 and that the XA21 intracellular domain is translocated to the nucleus in planta . Because XA21 does not carry a proline-rich domain indicative of intrinsic transcription activity, we hypothesized that the nuclear-localized XA21 interacts with transcription factors to control transcriptional reprogramming. To test this hypothesis, we assessed whether the rice transcription factor OsWRKY62, which negatively regulates XA21-mediated immunity [19] , interacts with the XA21 intracellular domain in plant cells. Indeed, using BiFC assays, we showed that the XA21 intracellular domain and OsWRKY62 interact exclusively in the nucleus of rice protoplasts ( Supplementary Fig. S8 ). XA21 kinase nuclear translocation is required for immune function We next assessed whether the nuclear localization of the XA21 intracellular domain is critical for XA21-mediated immunity. For this purpose, we generated transgenic rice plants expressing XA21 fused to a C-terminal nuclear export signal (NES) [20] ( Ubi -XA21-GFP-NES) and inoculated with Xoo ( Supplementary Fig. S9 ). Out of 12 independently transformed rice plants expressing Ubi-XA21-GFP-NES , all displayed significantly enhanced susceptibility to Xoo compared with the control transgenic rice plants expressing Ubi-XA21-GFP , lacking the NES. The NES did not affect the expression or stability of XA21-GFP ( Supplementary Figs S3b, S9a and S10 ). To quantify bacterial growth in the Ubi -XA21-GFP-NES lines, we measured lesion lengths and bacterial growth in the T 2 progeny using well-established techniques [14] ( Fig. 3 and Supplementary Fig. S11 ). At 4 days after inoculation (DAI), slight increases in the lesion lengths and bacterial populations were detected in the Ubi -XA21-GFP-NES lines compared with the Ubi -XA21-GFP control. At 12 DAI, the Ubi -XA21-GFL-NES displayed significantly enhanced susceptibility to Xoo , with lesions of approximately 10–13 cm. In contrast, the Ubi -XA21-GFP control displayed lesion lengths of 2–3 cm ( Fig. 3a ). The bacterial growth curve correlated well with lesion lengths ( Fig. 3b ). At 12 DAI, Xoo populations in Ubi -XA21-GFP transgenic rice reached approximately 7.8×10 7 colony-forming units (c.f.u.) per leaf (cfu/leaf), whereas populations in Kitaake plants reached to more than 3.6×10 9 c.f.u./leaf. In Ubi -XA21-GFP-NES line 7–22, Xoo populations grew to 1.2×10 9 c.f.u./leaf, a greater than 15-fold increase compared with the Ubi -XA21-GFP control. In Fig. 3c , we show two typical leaves from each of the inoculated rice plants at 12 days after Xoo inoculation. These results demonstrate that the nuclear translocation of the XA21 intracellular domain is required for its immune function. Rice plants expressing XA21-GFP-NES under the control of its native promoter ( Native -XA21-GFP-NES) were also susceptible compared with resistant Native -XA21-GFP, lacking NES ( Supplementary Fig. S12 ). These results demonstrate that nuclear translocation of the XA21 intracellular domain is required for XA21-mediated immunity. 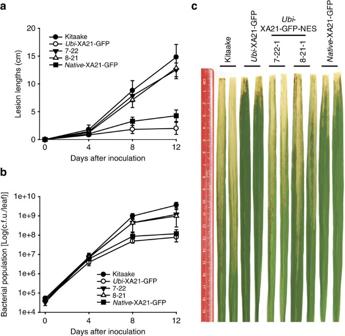Figure 3: Nuclear export of XA21 disrupts XA21-mediated immunity. (a) Lesion length measurements ofXoo-inoculated Kitaake,Ubi-XA21-GFP (homozygous 5-5-4),Ubi-XA21-GFP-NES (progeny from 7-22 and 8-21) orNative-XA21-GFP (progeny from 9 to 7) rice plants. Each data point represents the average and standard deviation of at least four samples. (b)Xoopopulations were monitored in Kitaake,Ubi-XA21-GFP (homozygous 5-5-4),Ubi-XA21-GFP-NES (progeny from 7 to 22 and 8-21) orNative-XA21-GFP (progeny from 9 to 7) rice plants. For each time point, bacterial populations were determined in three separate leaves for each genotype. Capped vertical bars represent standard deviation values (c.f.u./leaf) obtained from the three samples. (c) Transgenic plants expressing XA21 carrying a nuclear export signal (Ubi-XA21-GFP-NES) developed long lesion lengths afterXooinoculation. Rice leaves were photographed 12 days after inoculation (DAI) withXoo. From left to right: Kitaake,Ubi-XA21-GFP (homozygous 5-5-4),Ubi-XA21-GFP-NES (7-22-1 and 8-21-1) andNative-XA21-GFP (9-7-2) rice plants. Figure 3: Nuclear export of XA21 disrupts XA21-mediated immunity. ( a ) Lesion length measurements of Xoo -inoculated Kitaake, Ubi -XA21-GFP (homozygous 5-5-4), Ubi -XA21-GFP-NES (progeny from 7-22 and 8-21) or Native -XA21-GFP (progeny from 9 to 7) rice plants. Each data point represents the average and standard deviation of at least four samples. ( b ) Xoo populations were monitored in Kitaake, Ubi -XA21-GFP (homozygous 5-5-4), Ubi -XA21-GFP-NES (progeny from 7 to 22 and 8-21) or Native -XA21-GFP (progeny from 9 to 7) rice plants. For each time point, bacterial populations were determined in three separate leaves for each genotype. Capped vertical bars represent standard deviation values (c.f.u./leaf) obtained from the three samples. ( c ) Transgenic plants expressing XA21 carrying a nuclear export signal ( Ubi -XA21-GFP-NES) developed long lesion lengths after Xoo inoculation. Rice leaves were photographed 12 days after inoculation (DAI) with Xoo . From left to right: Kitaake, Ubi -XA21-GFP (homozygous 5-5-4), Ubi -XA21-GFP-NES (7-22-1 and 8-21-1) and Native -XA21-GFP (9-7-2) rice plants. Full size image The XA21 intracellular domain carries a functional nuclear localization sequence Many animal receptor kinases, including ErbB-4, Notch1 and β-amyloid precursor protein, undergo proteolytic cleavage by membrane-anchored proteases [21] , [22] , [23] . The released intracellular domains often carry a basic amino acid-rich nuclear localization sequence (NLS) [21] , [24] , [25] , XA21 also harbours a putative NLS in the intracellular domain ( Supplementary Fig. S13a ). To assess whether the putative XA21 NLS is functional, we investigated the cellular distribution of the XA21 intracellular domain. For this purpose, we generated a C-terminal GFP-tagged XA21 intracellular domain constructs containing a putative NLS ( XA21NLS-GFP ), a nonfunctional NLS with alanine substitutions ( XA21nls-GFP ), or a deletion of the putative NLS ( XA21NLS-GFP ) ( Supplementary Fig. S13a ). Whereas wild-type XA21NLS primarily localizes to the nucleus, alanine substitutions in the predicted NLS (XA21nls) or deletion of the NLS (XA21NLS) prevent XA21 nuclear localization ( Supplementary Fig. S13b ). These results suggest that the basic amino acid-rich region of the XA21 intracellular domain functions as an NLS. Whole plant studies with a full-length XA21 carrying a mutation in the NLS are needed to confirm this result. This study demonstrates that nuclear translocation of the XA21 intracellular domain is required for XA21-mediated immunity. Whereas C-terminal-tagged XA21 is primarily localized to the plasma membrane in the absence of AxY S 22 treatment with biologically active AxY S 22 or with supernatants prepared from Xoo triggers significant accumulation of XA21 inside the nucleus. We hypothesize that chaperone proteins may also be involved in the nuclear translocation of XA21. In support of this hypothesis, we have previously shown that the co-chaperones, RAR1 and SGT1, interact with the XA21 kinase domain in yeast and plant cells [26] . The HSP90/RAR1/SGT1 chaperone complex has previously been demonstrated to regulate the plant immune response [27] , [28] . These proteins are localized in both the cytoplasm and the nucleus, shuttling between these two compartments [28] , [29] , [30] , [31] . The observation that the non-RD kinase domain of a plant immune receptor is cleaved and localized to the nucleus where it interacts with a transcriptional regulator has not previously been reported. However, studies of animal TLRs and their associated non-RD kinases have demonstrated a similar nuclear localization requirement for activation of TLR-mediated immune responses. For example, on challenge with lipopolysaccharide or interleukin-1, IRAK1 localizes to the nucleus and binds to nuclear factor-κB-responsive elements located within the inhibitor of κB (IκB) -α promoter to regulate I κ B -α transcription [32] , [33] , [34] , [35] . Nuclear-localized IRAK1 also binds to the promoters of STAT3 and interleukin-10 upon lipopolysaccharide challenge and subsequently regulates interleukin-10 gene expression [34] , [36] . Together these results suggest a model for function of non-RD kinases associated with immune receptors. On receptor recognition of conserved microbial signatures, the associated non-RD kinase translocates to the nucleus where it directly interacts with transcription factors to regulate the immune response. Plant material and growth conditions Rice ( Oryza sativa L) plants (cultivar Kitaake) were maintained in the green house. Growth chambers were set on 14 h light/10 h dark photoperiod, 28/26 °C temperature cycle, and 85/90% humidity. Healthy and well-expanded leaves from 6-week-old rice plants were used for Xoo strain PXO99 inoculation (designated Xoo in text). Plasmid constructs Construction of Ubi -pCAMBIA-1300 has been described before [37] . For construction of XA21 driven by the XA21 native ( Native ) promoter, a 2,204-nt fragment from the XA21 promoter was amplified from rice genomic DNA extracted from Native -XA21 [18] transgenic plants using the following primers: 5′-AAGCTTGGTACCCAACTTTTTGTGCTCCTA-3′ and 5′-GGATCCCGTGCAGAAGTGCAAGGCAAGACA-3′. This construct was named XA21-pCAMBIA-1300. The XA21 promoter, was replaced with the maize ubiquitin ( Ubi ) constitutive promoter [38] using Hin dIII and Bam HI enzymes to generate the Ubi -pCAMBIA-1300 construct. The NES was generated by annealing the following oligonucleotides: 5′-GAACGAGCTTGCTCTTAAGTTGGCTGGACTTGATATTAACAAGACTGGAGGATAGCCCGGGCTGCA-3′ and 5′-GCCCGGGCTATCCTCCAGTCTTGTTAATATCAAGTCCAGCCAACTTAAGAGCAAGCTCGTTCTGCA-3′, encoding the amino-acid residues LQNELALKLAGLDINKTGG (stop) [20] . To amplify the XA21-GFP-Pst I site, PCR was performed using an XA21 -specific oligonucleotide primer and a GFP -specific oligonucleotide primer, 5′-CACCATGATATCACTCCCATTATTGCTC-3′/5′-CTGCAGTTTGTATAGTTCATCCATGCC-3′. Using PCR, the termination codon of XA21-GFP was replaced with Pst I site. The PCR-amplified products were cloned into pENTR/D-TOPO/D vector (Invitrogen). To generated XA21-GFP-NES , NES fragment was ligated into Pst I-digested XA21-GFP in pENTR/D-TOPO vector. Using Gateway LR Clonase (Invitrogen), XA21-GFP-NES and XA21-GFP moved into the Ubi -pCAMBIA-1300 (ref. 37 ) and Native -CAMBIA-1300. The XA21NLS-GFP was PCR amplified using oligonucleotides, 5′-CACCATGCACAAGAGAACTAAAAAGGGA-3′/5′-TTATTTGTATAGTTCATCCATGCCATG-3′ and template Ubi-XA21-GFP . The XA21nls-GFP and XA21 Δ NLS variants were amplified using oligonucleotides, 5′-CACCATGACCTGGGCAGCCGCAACTGCGGCAGGAGCCCCTTCAAGAACTTCCATGAAA-3′ and 5′-CACCATGGGAGCCCCTTCAAGAACTTCCATGAAA-3′, respectively. The PCR-amplified products were cloned into pENTR/D-TOPO vector. Using Gateway LR Clonase XA21NLS-GFP , XA21nls-GFP and XA21 Δ NLS moved into the Ubi -pCAMBIA-1300 (ref. 37 ). Rice transformation Rice transformation was constructed as described previously [37] . Agrobacterium strain EHA105 was used to infect rice callus from cultivar Kitaake for transformation. Transgenic lines were selected using hygromycin. Expression analysis. For reverse transcriptase-PCR (RT–PCR) analysis, total RNAs were extracted from leaves using TRIzol reagent (Invitrogen) after each treatment. The RT–PCR reaction was performed following the manual for QuantumRNA 18S Internal Standards (Ambion). PCR analyses were performed with primers pairs, 5′-TCATCACTCTACTTGCTTATA-3′/5′-TCAGAATTCAAGGCTCCCACCTTC-3′ (for XA21-GFP ). The amplified products were resolved by gel electrophoresis after 28 cycles. In vivo immunoprecipitation of XA21 Immunoprecipitation was conducted as described previously [16] . Total proteins were extracted from 5 g of leaf tissue in 25 ml of ice-cold extraction buffer II (0.15 M NaCl, 0.01 M Na-phosphate pH 7.2, 2 mM EDTA, 1% Triton X-100, 10 mM β-mercaptoethanol, 20 mM NaF, 1 mM phenylmethylsulphonyl fluoride, 1% protease cocktail (Sigma), 2 mg ml −1 leupeptin, 2 mg ml −1 antipain and 2 mg ml −1 aprotinin). After filtering through Miracloth (Calbiochem) followed by centrifugation twice at 13,000 g for 20 min at 4 °C, the supernatant was mixed with 50 ml of agarose-conjugated anti-Myc antibody (Santa Cruz) for Myc-XA21 and anti-GFP antibody (Santa Cruz) for XA21-GFP and incubated at 4 °C for 2 h. The beads were then washed four times in 1 ml of extraction buffer II without proteinase inhibitors. The proteins were eluted with 4× Laemmli-loading buffer. Protein blot analyses were performed. Immunodetection For immunoblot analysis, proteins were separated by an 8% SDS–polyacrylamide gel. The proteins were then blotted onto a Hybond-P membrane (Amersham Pharmacia Biotech) using a SemiPhor Semi-Dry Transfer Unit (Amersham Pharmacia Biotech). For XA21-GFP detection, anti-GFP mouse monoclonal IgG (Santa Cruz) and anti-mouse IgG, horseradish peroxidase-linked whole antibody were used as primary and secondary antibodies at a final dilution of 1:1,000 and 1:5,000 for 2 h, respectively. Bands were visualized using the SuperSignal West Pico Chemiluminescent Substrate (Pierce) according to standard protocol. For the anti-XA21 kinase and XA21 LRR antibodies, synthetic peptides and monospecific antibodies were generated. Epitope selection was directed to hydrophobic, flexible regions of the proteins. The epitopes, RNLFQTREQDDWGFI in the LRR domain and KALKSFTAECEALRN in the kinase domain were used for anti-XA21 LRR and XA21 kinase antibodies, respectively. Peptides were synthesized and conjugated to keyhole limpet haemocyanin. Rabbits were immunized with peptide in complete Freund's adjuvant, followed by three boosts in incomplete Freund's adjuvant. Monospecific antibodies were affinity-purified to the synthetic peptides bound to C3-SEP-PAK cartridges. Antibodies were conjugated to horseradish peroxidase for use in western blots. Xoo inoculation and determination of bacterial populations For Xoo inoculation, rice plants were grown in the greenhouse until they were 6-week-old and then transferred to the growth chamber. Xoo was used to inoculate rice by the scissors-dip method [14] , [37] . Xoo was grown on a PSA plate (peptone sucrose agar, 10 g l −1 peptone, 10 g l −1 sucrose, 1 g l −1 glutamic acid, 16 g l −1 agar and pH 7.0) containing cephalexin (100 μg l −1 ) for 3 days and suspended with water at OD=0.5 (600 nm) for inoculation. Only the top two to three expanded leaves of each tiller were inoculated. Xoo colony count was conducted as described previously [14] , [16] , [37] . Twenty centimeter of leaf tissue from the top, including lesions and tissue showing no lesions, was ground up and resuspended in 10 ml water to collect bacteria. The extract was diluted accordingly and plated out on PSA plates. Xoo and AxY S 22 treatments of rice leaf discs Leaf disc assays [39] were modified for Xoo and AxY S 22 treatments of rice. Briefly, fully expanded rice leaves were shredded into 2–3 mm with scissors. Because previous studies have demonstrated that leaf discs floated overnight do not show symptoms of wounding [39] , [40] , [41] , the shredded leaves were floated and maintained in a growth chamber under 14 h light/10 h dark conditions with 28 °C for 1 day to recover from wounding. After 3 h incubation with 1 μM AxY S 22, 1 μM AxY22 or Xoo (OD=0.5 at 600 nm), the shredded leaves were immediately frozen in liquid nitrogen for protein extractions. Nuclei isolation Nuclear fractionation was performed using CellLytic PN Plant Nuclei Isolation/Extraction Kit (Sigma) with minor modifications. Briefly, tissue was homogenized in 1× nuclear isolation buffer (NIB) containing 1 mM DTT and protease inhibitor cocktail for plant cell (Sigma) using a mortar and pestle and then filtered through a 100-μm (pore-size) nylon mesh. Triton X-100 was added to a final concentration of 1.0%, and the mixture was incubated on ice for 15 min. The solution was centrifuged at 12,000 g for 10 min, and the pellet was washed with 1× NIB containing 1 mM DTT and protease inhibitor cocktail. Nuclei-containing lysate was applied to 1.7 M sucrose cushion and centrifuged at 12,000 g for 10 min. Nuclei pellet was washed twice with 1× NIB containing 1 mM DTT and protease inhibitor cocktail and stored in nuclei storage buffer (Sigma). XA21-GFP and XA21-GFP-NES transient expression analyses Plasmids, Ubi-XA21-GFP , Ubi-XA21-GFP-NES , XA21NLS-GFP , XA21nls-GFP and XA21NLS-GFP driven by Ubi promoter [38] , were used for transient expression analyses. Images were collected with a Leica True Confocal Scanner SPE confocal microscope. GFP was imaged under the following conditions: excitation, 488 nm and emission, 500–530 nm. DsRed was imaged under the following conditions: excitation, 532 nm and emission, 560–620 nm. Images were analysed using Leica LAS AF software (Ver 2.3.5) and coded green (for GFP) or red (for DsRed). BiFC assays Plasmids, 735-YFP C−term (YC)-XA21K668, 736-YFP N−term (YN)-OsWRKY62 and Ubi -YFP, were described previously [26] . As negative controls, we included the both empty vectors (735-YC-empty vector and 736-YN-empty vector) for each pairwise test. All images were taken 1 day after transformation. Yellow fluorescent protein (YFP) was imaged under the following conditions: excitation, 488 nm and emission, 515–565 nm. Images were analysed using Leica LAS AF software (Ver 2.3.5) and coded yellow for YFP. How to cite this article: Park, C.-J. & Ronald P.C. Cleavage and nuclear localization of the rice XA21 immune receptor. Nat. Commun. 3:920 doi: 10.1038/ncomms1932 (2012).